Twisted optical metamaterials for planarized ultrathin broadband circular polarizers Optical metamaterials are usually based on planarized, complex-shaped, resonant nano-inclusions. Three-dimensional geometries may provide a wider set of functionalities, including broadband chirality to manipulate circular polarization at the nanoscale, but their fabrication becomes challenging as their dimensions get smaller. Here we introduce a new paradigm for the realization of optical metamaterials, showing that three-dimensional effects may be obtained without complicated inclusions, but instead by tailoring the relative orientation within the lattice. We apply this concept to realize planarized, broadband bianisotropic metamaterials as stacked nanorod arrays with a tailored rotational twist. Because of the coupling among closely spaced twisted plasmonic metasurfaces, metamaterials realized with conventional lithography may effectively operate as three-dimensional helical structures with broadband bianisotropic optical response. The proposed concept is also shown to relax alignment requirements common in three-dimensional metamaterial designs. The realized sample constitutes an ultrathin, broadband circular polarizer that may be directly integrated within nanophotonic systems. Circular dichroism, bianisotropy and magneto-electric coupling, found in chiral molecules, are at the origin of the different optical response of natural materials to left-handed (LCP) and right-handed circularly polarized (RCP) excitations. On the basis of these concepts, three-dimensional (3D) chiral structures such as helices may be used to realize circular polarizers [1] , [2] . Similarly, cholesteric liquid crystals are composed of chiral molecules with a helical pitch that may be used to selectively filter one circular polarization based on Bragg reflection [3] , [4] , [5] , [6] . Conventional circular polarizers based on these concepts typically operate over narrow frequency bands [4] , which may be broadened by stacking multiple polarizers or introducing a gradient in the helical pitch [3] , [6] . However, modest bandwidth increases are usually achieved at the price of much bulkier devices, which are difficult to integrate within today's nanophotonic systems. Recent advances in metamaterials [3] , [7] , [8] , [9] , [10] , [11] have opened new routes towards integrated circular polarizers with low-profile and larger bandwidths of operation. In part inspired by biological species that are well equipped with broadband, conformal circular polarization sensors [12] , optical activity and circular dichroism have been shown in either planar [13] , [14] , [15] , [16] , [17] , [18] or three-dimensional metamaterials [3] , [19] , [20] . Planar structures generally exhibit much weaker circular dichroism compared with 3D geometries, because an infinitesimally thin device is inherently achiral, and excitation at oblique incidence or some form of nonreciprocal response is required to distinguish between LCP and RCP transmissivity [21] . In this context, the concept of extrinsic chirality has been recently put forward, showing that, by pairing two closely spaced planarized inclusions with some form of 3D chirality, may produce a narrow-band chiral response near their resonance [13] , [14] , [15] , [16] , [17] , [18] . 3D chiral metamaterials have more appealing properties as circular polarizers, but periodic arrays with subwavelength chiral features and precise alignment are challenging to realize at visible wavelengths, despite several available top-down [3] and bottom-up [19] fabrication approaches. An exciting possibility in this context is provided by direct laser writing [22] , [23] , which ensures large flexibility in the shape of the realizable 3D metamaterial inclusions. Broadband infrared circular polarizers based on gold helical metamaterials [1] have been recently demonstrated using this technique; however, realizing these structures in the visible is hindered by the minimum realizable features imposed by the diffraction limit. We propose here an alternative venue to realize strong, broadband bianisotropic effects in metamaterials, not based on chirality at the inclusion level, but instead on the relative orientation of strongly anisotropic achiral surfaces, introducing and applying the concept of twisted metamaterials. Our design is based on stacked planar metasurfaces realized with conventional lithographic techniques, suitably rotated from one layer to the next. Our goal is to show that, by introducing a twist in the lattice orientation of metamaterial inclusions, we can relax the usual requirements on fabrication and achieve exotic effects analogous to 3D metamaterials, but with much simpler fabrication schemes. In this context, it has been recently shown at microwave frequencies [18] that broadband linear polarization conversion may be obtained by coupling together twisted magnetic inclusions. Here we show that broadband circular polarization selectivity may be achieved in twisted arrays of metasurfaces without the need of complicated inclusion shape, with no requirement on the relative alignment, and at optical frequencies. We use a generalized Bloch analysis to model the cascaded structure [24] , in combination with optical transmission-line theory [25] , and show that this concept may relax several constraints in the realization of 3D bianisotropic metamaterials, including inclusion shape requirements and lateral alignment between neighbouring inclusions. Concept and optimized design of twisted metamaterials Consider first a single plasmonic metasurface made of gold [26] nanorods, with thickness t =50 nm, periods d x =300 nm, d y =300 nm, length l =250 nm and width w =60 nm. The shape of the nanorods is chosen to produce strong, resonant anisotropy within the plane, but it is strictly achiral. Because of the subwavelength thickness t , LCP and RCP transmissivities are expected to be identical for normal incidence at all frequencies. This may be readily proven by modelling the metasurface with its equivalent anisotropic shunt admittance Y s (ref. 27 ), which relates the averaged tangential polarization currents J s to the total tangential electric field E tot on the surface producing a discontinuity in the total tangential magnetic fields H tot on the array plane z =0. By considering the reciprocity requirement where the superscript T denotes transpose, it follows that LCP and RCP transmissivities are bound to be equal [28] : A small cross-coupling component T LR = T RL also arises, but it is not relevant to the following discussion. To convert the strong surface anisotropy around the nanorod resonance into chiral bianisotropy, we consider cascading two identical metasurfaces with a subwavelength separation distance L and a specific rotation angle θ of the second surface compared with the first one ( Fig. 1a ). In this context, 3D chiral inclusions have been obtained by pairing two strongly coupled 2D chiral planar particles [17] , rotated one with respect to the other, based on the concept of extrinsic chirality. We consider here completely achiral inclusions (simple nanorods) forming strongly anisotropic arrays, with the aim of converting their anisotropy into magneto-electric coupling by rotation, as a pure lattice effect. As discussed in ref. 27 , our transmission-line model may be successfully applied to model this configuration, as sketched in the circuit model of Fig. 1i , which includes a transmission-line segment to model each gap between neighbouring metasurfaces and the rotation matrix describing the relative rotation of the second impedance tensor compared with the first one In this scenario, T LL and T RR through the stack are no longer bound to have the same magnitude and, using our analytical model, we are able to conveniently assess the predicted circular polarization properties of the metasurface pair by calculating the extinction ratio | T RR / T LL | at each wavelength as a function of L and θ . Figure 2a shows, as an example, the wavelength dispersion of | T LL | and | T RR | for L =120 nm and θ =60°. 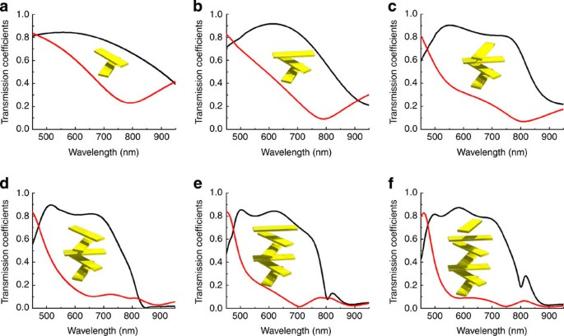Figure 2: Evolution of the frequency response by increasing the number of stacks. Transmission of LCP and RCP waves through a stack of rotated metasurfaces by increasing the number of layers (L=120 nm,θ=60°). In (a–f), the number of layers increases from two to seven, with the insets illustrating one unit cell of the corresponding twisted metamaterial slab along the direction of propagation. A right-handed rotation of the second array with respect to the first one produces preferential transmission of RCP waves, with maximum separation near the array resonance, spanning over a moderate wavelength range (~700 nm). We define the circular polarizer bandwidth of this pair as the span of wavelengths over which the extinction ratio is larger than for clockwise rotation 0< θ <90°. In Fig. 1 , we show the calculated bandwidth ( Fig. 1b ), the corresponding average extinction ratio | T RR / T LL | ( Fig. 1c ) and the overall figure of merit (FoM, Fig. 1d ), defined as the product of bandwidth and extinction ratio, as a function of L and θ . It is seen that optimal performance is obtained for subwavelength separation distances and for a rotation angle around θ ~60°. We did not consider here distances smaller than 80 nm, because our analytical model neglects higher order Floquet modes in the coupling between neighbouring metasurfaces, losing its accuracy for smaller distances. In any case, it is found that the optimal distance is in the range L ~150 nm, and closer metasurfaces cannot achieve as large FoM. 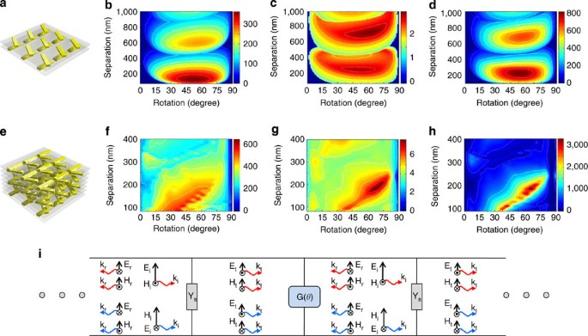In this range, we have verified that our analytical results match very well with full-wave simulations of the pair. Figure 1: Circular polarization selectivity of twisted metamaterials. (a) Illustration of a pair of stacked metasurfaces with rotational twistθand separation distanced, together with (b) calculated bandwidth in nanometres, (c) extinction ratio, (d) and figure of merit, as defined in the text. (e) Illustration of a seven-layer twisted metamaterial, and corresponding (f) calculated bandwidth, (g) extinction ratio, (h) and figure of merit. (i) Transmission-line model, whereYsis the surface admittance of a single metasurface,G(θ) is the rotation matrix. Figure 1: Circular polarization selectivity of twisted metamaterials. ( a ) Illustration of a pair of stacked metasurfaces with rotational twist θ and separation distance d , together with ( b ) calculated bandwidth in nanometres, ( c ) extinction ratio, ( d ) and figure of merit, as defined in the text. ( e ) Illustration of a seven-layer twisted metamaterial, and corresponding ( f ) calculated bandwidth, ( g ) extinction ratio, ( h ) and figure of merit. ( i ) Transmission-line model, where Y s is the surface admittance of a single metasurface, G ( θ ) is the rotation matrix. Full size image Figure 2: Evolution of the frequency response by increasing the number of stacks. Transmission of LCP and RCP waves through a stack of rotated metasurfaces by increasing the number of layers ( L =120 nm, θ =60°). In ( a – f ), the number of layers increases from two to seven, with the insets illustrating one unit cell of the corresponding twisted metamaterial slab along the direction of propagation. Full size image Since a pair of achiral, anisotropic metasurfaces can support circular polarization selectivity over a moderately broad bandwidth after properly rotating one of them, it may be expected that, by stacking a larger number of closely spaced metasurfaces with sequential rotation, the FoM may increase, similar to the bandwidth increase in metamaterials formed by a large number of closely spaced resonant inclusions. We verify this possibility in Fig. 1e–h , in which we show analogous results for a stack of seven metasurfaces for fixed separation distance L and angle of rotation θ between any two consecutive elements, as in Fig. 1e . Indeed, it is seen that bandwidth, extinction ratio and overall FoM can dramatically increase by combining closely spaced metasurfaces with proper sequential rotation and period. This is indeed consistent with the way the bandwidth of metamaterials drastically increases compared with the resonance of their individual inclusions, provided that they are densely packed [29] . Optimal parameters are found in a similar range of L and θ , but with more selectivity in terms of their value for optimal performance. Functionality and operation To show how the bandwidth evolves when stacking metasurfaces with sequential rotation, we show in Fig. 2 the evolution of the transmission coefficients for L =120 nm and θ =60° when increasing the number of layers, as indicated in each inset. By cascading more layers, the bandwidth is gradually broadened, spanning nearly the entire visible range in the case of seven layers ( Fig. 2f ), with also a much increased extinction ratio. For a right-handed twist, LCP waves are reflected within the bandwidth of operation, whereas RCP is transmitted, consistent with the previous discussion. It appears that, by increasing the number of stacked metasurfaces, we are able to move from a simple resonant response to a continuous stop band, transitioning from a one-element filter to a homogeneous twisted metamaterial. In this regard, we have extended our analytical model to analyse the eigenmodal properties of this rotated stack for a number of layers N → ∞, considering the generalized Bloch eigenmodes supported in a suitable reference system that rotates with each successive layer, analogous to the approach used to analyse linear arrays of rotated particles [24] . Although the details of this homogenization theory for twisted metamaterials go beyond the focus of the present work, it is relevant to point out that we have verified how one of the two generalized eigenmodes supported by the homogenized twisted metamaterial, based on the parameters of Fig. 2 , is indeed characterized by purely LCP fields, and supports a continuous stop band spanning the visible range. This finding highlights the unique response of twisted metamaterials compared with extrinsic chirality or nematic liquid crystals: the subwavelength sequential rotation through the stack effectively transforms the strong resonant anisotropy of each metasurface into a unique form of broadband magneto-electric coupling, responsible for circularly polarized eigenmodes, sustained by the lattice rather than by the chirality of the individual inclusions. Period and twist angle of the stack can then be optimized to broaden and tune the stop band of one of them, to ensure the optimal operation as a circular polarizer. It should be stressed that the functionality of the twisted metamaterial slab introduced here is very distinct from cholesteric liquid crystals or helicoidal materials [30] , which also support circular polarization selectivity by sequential rotation of chiral molecules [4] . In those materials, the anisotropy of each layer is very weak, and the rejection of one circular polarization is obtained over several wavelengths based on Bragg reflection, under the condition that the helical pitch of the crystal is comparable to the wavelength of operation [5] . The operation of twisted metamaterials, on the contrary, is based on strong, resonant anisotropy at the metasurface level (without relying on chirality at all), which is broadened by the strong coupling among closely spaced surfaces, over a subwavelength period. The rotational pitch of the metamaterial considered in Fig. 2 , for instance, is about one-tenth of the one that would be required in a cholesteric liquid crystal to obtain some form of polarization selectivity, and we obtain here a much larger extinction ratio, across a subwavelength thickness, with much more broadband response. The rotational twist along the lattice adiabatically transforms linearly polarized eigenmodes, supported by resonant, anisotropic metasurfaces, into circularly polarized ones. The clearest differences between twisted metamaterials and cholesteric liquid crystals or helicoidal materials consist in the drastically larger bandwidth, associated with strong coupling among neighbouring metasurfaces, and the fact that cholesteric liquid crystals reflect the handedness associated with the helical rotation due to Bragg reflection, whereas the twisted metamaterial transmits that polarization, because its rotation over a subwavelength scale adiabatically rotates in the same direction as the eigenmodal polarization. Shift invariance and robustness to misalignments One additional advantage of the twisted metamaterial concept is its expected robustness to misalignments, which may be found in layer-by-layer fabrication. As the proposed concept is based on the metasurfaces coupled through the dominant transverse Floquet mode, and not on the individual inclusion resonant interaction with light, it is expected that arbitrary alignment between neighbouring layers should not affect the overall response of the twisted metamaterial. This is obviously drastically different from extrinsic chirality, which is inherently based on the strong coupling between neighbouring pairs of rotated inclusions. This is verified in Fig. 3 , where we show LCP and RCP transmission coefficients for a stack of seven layers, similar to Fig. 2f , considering different forms of misalignment, as indicated in Fig. 3b–d . When one of three consecutive metasurfaces is misaligned in one direction ( Fig. 3c ), or even when all of them are misaligned in both directions ( Fig. 3d ), still the same transmission curves, as in the ideally aligned case ( Fig. 3b ), are obtained. The total level of loss is slightly increased when misalignment and disorder is introduced, but without significantly affecting the performance of the device. 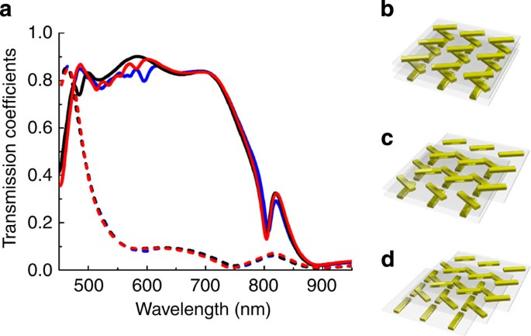Figure 3: Robustness to misalignment. (a) Three sets of transmission coefficients are presented, corresponding to (b) ideal alignment of three consecutive metasurfaces (black); (c) misalignment of one metasurface along one transverse direction (blue); (d) misalignment of all metasurfaces in the stack in both directions (red); solid curves refer to RCP, dashed curves to LCP. Figure 3: Robustness to misalignment. ( a ) Three sets of transmission coefficients are presented, corresponding to ( b ) ideal alignment of three consecutive metasurfaces (black); ( c ) misalignment of one metasurface along one transverse direction (blue); ( d ) misalignment of all metasurfaces in the stack in both directions (red); solid curves refer to RCP, dashed curves to LCP. Full size image Experimental realization and characterization We have verified the functionality of the proposed twisted metamaterial by realizing and characterizing several devices, going from one-layer to a four-layer stack. 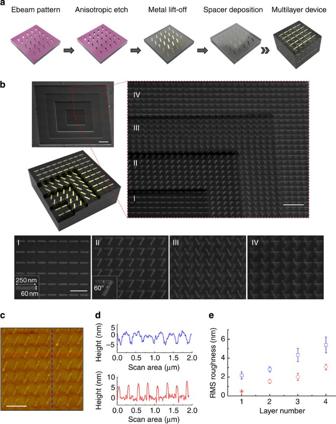Figure 4: Device fabrication. (a) Fabrication scheme to realize each layer of the twisted metamaterial. A multi-layer stack can be obtained after repeating the first four steps (see Methods). (b) Multilayer SEM view of the realized four-layer device. The images are prepared through focussed-ion beam milling to reveal each layer, where I, II, III, IV mark the corresponding layers. The inset in layer I shows the dimensions of each nanorod; the inset in layer II shows the measured rotation angle between adjacent layers. The sample was prepared by coating 5 nm of Pt/Pd before SEM imaging to reduce charging effect, due to the non-conducting nature of the silicon dioxide substrate. The scale bars in the SEM images from top to bottom are 2 μm, 1 μm, and 500 nm, respectively. (c) AFM image of a two-layer device and corresponding surface profile to measure the planarization: the first layer (horizontal rods) considers the planarization after metal lift-off and silicon dioxide spacer deposition (blue curve in (d)), the peak to valley height is within 5 nm; the second layer (60° tilted rods) is obtained after metal lift-off, but before silicon dioxide deposition (red curve in (d)), here the peak to valley height is within 7 nm. Scale bar in (c) is 500 nm. (e) Root mean square (RMS) surface roughness of each layer before (blue square) and after (red circle) silicon-dioxide deposition. Surface roughness is improved after silicon dioxide deposition. Figure 4a shows the relevant fabrication steps of our design, as described in more detail in the Methods. Our final fabricated sample consists of four planar arrays of gold nanorods, based on the design of Fig. 2 . Figure 4b shows the scanning electron microscope (SEM) images of the realized device, obtained using focussed-ion beam milling to reveal the details of each cascaded layer. The atomic force microscope (AFM) image and characterization in Fig. 4c–e shows the details of the planarization process that we applied to realize the cascaded structure, as described in the Methods. We have performed full-wave numerical simulations and experimental characterization of LCP and RCP transmissivities through the several stages of this device, going from a one-layer metasurface to the four-layer twisted metamaterial slab, sequentially stacking more metasurfaces. In our simulations, shown in Fig. 5a–d , we have included the dielectric spacers and titanium adhesion layers required for the realization of the twisted metamaterial (see fabrication details in the Methods), which were not considered in Fig. 2 . As predicted by simulations, their presence slightly shifts the operation of the twisted metamaterial to longer wavelengths, and contributes to additional absorption losses residing in the thin adhesion layers, which slightly reduces the bandwidth and FoM of the polarizer. Measured and simulated curves follow each other quite closely: the single metasurface ( Fig. 5e ) provides the expected identical transmission of LCP and RCP waves, but as soon as a second layer is cascaded with proper twist and distance ( Fig. 5f ), we obtain some form of polarization selectivity. As predicted by our theory, a larger number of layers ( Fig. 5g,h ) ensures better extinction ratios and increased bandwidths. Despite some unwanted absorption due to the nonideal fabrication conditions, the four-layer device operates as a broadband, ultrathin circular polarizer, consistent with the operation of a 3D bianisotropic metamaterial, confirming the functionality as a twisted metamaterial. Figure 4: Device fabrication. ( a ) Fabrication scheme to realize each layer of the twisted metamaterial. A multi-layer stack can be obtained after repeating the first four steps (see Methods). ( b ) Multilayer SEM view of the realized four-layer device. The images are prepared through focussed-ion beam milling to reveal each layer, where I, II, III, IV mark the corresponding layers. The inset in layer I shows the dimensions of each nanorod; the inset in layer II shows the measured rotation angle between adjacent layers. The sample was prepared by coating 5 nm of Pt/Pd before SEM imaging to reduce charging effect, due to the non-conducting nature of the silicon dioxide substrate. The scale bars in the SEM images from top to bottom are 2 μm, 1 μm, and 500 nm, respectively. ( c ) AFM image of a two-layer device and corresponding surface profile to measure the planarization: the first layer (horizontal rods) considers the planarization after metal lift-off and silicon dioxide spacer deposition (blue curve in ( d )), the peak to valley height is within 5 nm; the second layer (60° tilted rods) is obtained after metal lift-off, but before silicon dioxide deposition (red curve in ( d )), here the peak to valley height is within 7 nm. Scale bar in ( c ) is 500 nm. ( e ) Root mean square (RMS) surface roughness of each layer before (blue square) and after (red circle) silicon-dioxide deposition. Surface roughness is improved after silicon dioxide deposition. 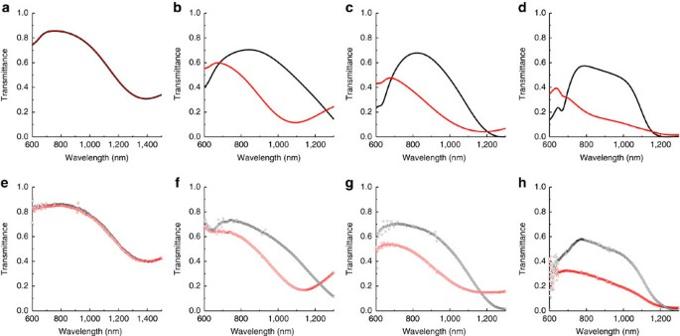Figure 5: Comparison between measurements and simulations. (a–d) Full-wave numerical simulations for twisted metamaterial slabs with 1 to 4 layers. Black lines are for RCP and red lines are for LCP transmission. As predicted by theory and simulations, the bandwidth and extinction ratio is increased with a larger number of layers of the twisted metamaterial. (e–h) Corresponding experimental measurements, where black circles represent RCP and red triangles represent LCP transmission; the measurement is obtained by scanning the wavelength with a resolution of 2 nm as described in the Methods. Full size image Figure 5: Comparison between measurements and simulations. ( a – d ) Full-wave numerical simulations for twisted metamaterial slabs with 1 to 4 layers. Black lines are for RCP and red lines are for LCP transmission. As predicted by theory and simulations, the bandwidth and extinction ratio is increased with a larger number of layers of the twisted metamaterial. ( e – h ) Corresponding experimental measurements, where black circles represent RCP and red triangles represent LCP transmission; the measurement is obtained by scanning the wavelength with a resolution of 2 nm as described in the Methods. Full size image Chiral bianisotropy, purely based on a lattice effect, has been obtained using an array of purely three-dimensionally achiral inclusions, realized with standard lithographic techniques and planarized technology. We believe that with a similar technique it may be possible to realize broadband circular polarizers at even shorter wavelengths, spanning the entire visible range, and reduce the amount of losses by avoiding lossy metals for the adhesion layers and considering lower-loss plasmonic materials for the nanorods, for example, silver. The proposed broadband circular polarizers may be directly integrated into nanophotonic devices, because of its ultralow and planar profile. Our proposed concept may be easily scaled up to longer wavelengths for a variety of exciting applications in the mid-infrared and terahertz spectral range, for which convenient sources, such as quantum cascade lasers, are available, but advanced optical elements for polarization control such as achromatic quarter wave plates or broadband circular polarizers are currently unavailable. More broadly, we believe that the proposed concept of twisted metamaterials, obtained by breaking the periodicity of conventional metamaterials by introducing a sequential twist within the lattice, may broaden the venues in which optical metamaterials may be realized and applied, by relaxing several of the requirements on the inclusion shape. This may have groundbreaking impact in a variety of novel metamaterial devices and applications, beyond polarization manipulation and control, for example, in tailoring spatial dispersion or modal propagation. We are currently exploring some of these venues. Device fabrication The fabrication stages are shown in Fig. 4a . Gold alignment marks 100 nm thick were first fabricated on bare glass substrate (C1737-0107, Delta Technologies), then 100 nm silicon dioxide was deposited on the substrate using e-beam evaporator. E-beam resist ZEP 520 was first diluted with ZEP A (Anisole), then spun onto the substrate to obtain a thickness of 100 nm. The pattern was written using a JBX-6000FS/E e-beam aligner at an accelerating voltage of 50 kV. After exposure, the sample was developed in ZED-N50 (Emyl Acetate). The pattern was then transferred to the silicon dioxide thin film by reactive ion etching using a gas mixture of CF 4 and helium in Trion Oracle plasma etcher to etch off 55 nm of silicon dioxide. A 5-nm titanium adhesion layer and 50 nm gold were sequentially deposited onto the sample using CHA e-beam evaporator. Then, the sample underwent the lift-off process in N -methyl-2-pyroridone to complete the first layer. 100 nm silicon dioxide layer served as a dielectric spacer, coated through e-beam evaporation. The surface was automatically planarized after metal lift-off. A special effort was made to ensure flat surface after each metal nanorod deposition. To achieve this, the metal lift-off e-beam resist mask was first used to etch 55-nm-deep trenches in the substrate via reactive ion etching; a 55-nm thick metal layer was then deposited. After the lift-off process, the metal nanorods are positioned in the trenches etched in the substrate. The AFM image in Fig. 4c–e shows the planarization measurement of each layer before and after the deposition of a silicon dioxide spacer. The planarization process reduced surface-height variation from 55 nm to 5 nm. Subsequent layers were added by repeating similar steps, from silicon dioxide deposition to metal lift-off. Optical measurements Testing was conducted after processing each layer. To test the resonance of a single layer, a halogen broadband light source was coupled into a spectrograph (Princeton instrument SpectraPro-2500i) to scan the wavelength with a resolution of 2 nm. The output light from the spectrograph was sequentially passed through a linear polarizer (Thorlabs LPVIS050), a broadband quarter-wave plate (Thorlabs AQWP05M-980), the sample, a second broadband quarter-wave plate, a second linear polarizer, and finally an InGaAs detector (Princeton instrument Model ID441-C). How to cite this article: Zhao, Y. et al . Twisted optical metamaterials for planarized ultrathin broadband circular polarizers. Nat. Commun. 3:870 doi: 10.1038/ncomms1877 (2012).